Sulfhydration mediates neuroprotective actions of parkin Increases in S-nitrosylation and inactivation of the neuroprotective ubiquitin E3 ligase, parkin, in the brains of patients with Parkinson’s disease are thought to be pathogenic and suggest a possible mechanism linking parkin to sporadic Parkinson’s disease. Here we demonstrate that physiologic modification of parkin by hydrogen sulfide, termed sulfhydration, enhances its catalytic activity. Sulfhydration sites are identified by mass spectrometry analysis and are investigated by site-directed mutagenesis. Parkin sulfhydration is markedly depleted in the brains of patients with Parkinson’s disease, suggesting that this loss may be pathologic. This implies that hydrogen sulfide donors may be therapeutic. Parkin is an E3 ubiquitin ligase that ubiquitinates diverse substrates [1] . Mutations in parkin, which disrupt its catalytic activity, are the most common cause of autosomal recessive Parkinson’s disease (PD), indicating that loss of parkin is neurotoxic, whereas its enhancement is neuroprotective [1] , [2] . Parkin may also participate in the pathophysiology of the much more common sporadic form of PD based on interactions with nitric oxide (NO). Dawson and colleagues [3] and Lipton and colleagues [4] reported that parkin is S-nitrosylated with greatly increased nitrosylation in brains of patients with PD. Nitrosylation of parkin inhibits its E3 ligase and neuroprotective activities, implying that the increased nitrosylation of parkin in PD is pathogenic. Recently, hydrogen sulfide (H 2 S) has been appreciated as a gasotransmitter comparable to NO and CO [5] , [6] , [7] , [8] . H 2 S signals primarily by attaching to SH groups of cysteines in proteins, a process termed sulfhydration [9] . Sulfhydration generally occurs on the same cysteines as nitrosylation so that the two processes may be reciprocal. This prompted us to explore relative roles of sulfhydration and nitrosylation in the function of parkin. We report that parkin is physiologically sulfhydrated and that, whereas nitrosylation inactivates parkin, sulfhydration stimulates its activity. We identify major declines of parkin sulfhydration in the corpus striatum of PD patients. We also show that H 2 S donors are cytoprotective in PD-related models of neurotoxicity. Thus, diminished sulfhydration of parkin may be pathogenic in PD and selective H 2 S donors may be therapeutic. Parkin is physiologically sulfhydrated The biotin switch method that we developed [10] for monitoring nitrosylation can be modified to identify sulfhydration [9] . Utilizing the modified biotin switch assay, we demonstrate sulfhydration of overexpressed parkin in response to treatment with the H 2 S donor NaHS ( Fig. 1a ). Recently, we have developed improved methodology for monitoring sulfhydration, by employing fluorescently labelled derivatives of maleimide [11] . Virtues of the maleimide procedure include its greater specificity, the ability to quantify results readily and the capacity of the technique to monitor nitrosylation and sulfhydration of the same samples [11] . Using the maleimide procedure, we establish that under basal conditions parkin is robustly sulfhydrated in whole brain of mice and the striatum of rats ( Fig. 1b ). 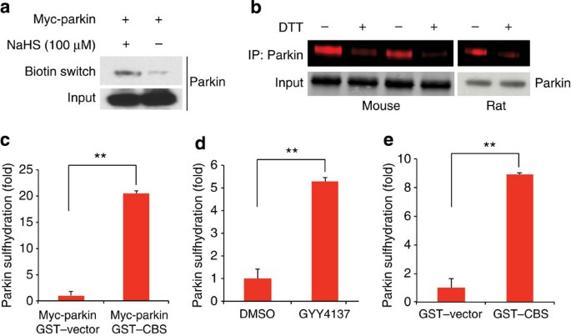Figure 1: Parkin is physiologically sulfhydrated. (a) Parkin expressed in HEK293 cells is sulfhydrated by the H2S donor NaHS as detected by the modified biotin switch method. (b) Endogenous parkin is basally sulfhydrated in both mouse brain and rat striatum as detected by the maleimide assay, in which loss of red fluorescence signal following DTT treatment indicates sulfhydration of the protein. (c) Sulfhydration of myc-parkin overexpressed in HEK293 cells is enhanced almost 20-fold on overexpression of GST–CBS, one of the principle H2S producers in the brain.n=3, **P<0.01 via one-way analysis of variance (ANOVA). (d) Endogenous parkin sulfhydration in SH-SY5Y cells is enhanced over fivefold on treatment with 100 μM GYY4137, a hydrogen sulfide donor.n=3, **P<0.01 via one-way ANOVA. (e) Endogenous parkin sulfhydration in SH-SY5Y cells is enhanced over eightfold by overexpression of GST–CBS.n=3, **P<0.01 via one-way ANOVA. All data are expressed as mean±s.e.m. Figure 1: Parkin is physiologically sulfhydrated. ( a ) Parkin expressed in HEK293 cells is sulfhydrated by the H 2 S donor NaHS as detected by the modified biotin switch method. ( b ) Endogenous parkin is basally sulfhydrated in both mouse brain and rat striatum as detected by the maleimide assay, in which loss of red fluorescence signal following DTT treatment indicates sulfhydration of the protein. ( c ) Sulfhydration of myc-parkin overexpressed in HEK293 cells is enhanced almost 20-fold on overexpression of GST–CBS, one of the principle H 2 S producers in the brain. n =3, ** P <0.01 via one-way analysis of variance (ANOVA). ( d ) Endogenous parkin sulfhydration in SH-SY5Y cells is enhanced over fivefold on treatment with 100 μM GYY4137, a hydrogen sulfide donor. n =3, ** P <0.01 via one-way ANOVA. ( e ) Endogenous parkin sulfhydration in SH-SY5Y cells is enhanced over eightfold by overexpression of GST–CBS. n =3, ** P <0.01 via one-way ANOVA. All data are expressed as mean±s.e.m. Full size image To further substantiate the nature of parkin sulfhydration, we show that overexpression of cystathionine β-synthase (CBS), an H 2 S biosynthetic enzyme, increases parkin sulfhydration more than 20-fold ( Fig. 1c and Supplementary Fig. S1a ). The neuronal cell line SH-SY5Y displays endogenous sulfhydration of parkin, which is increased more than fivefold by treatment with the H 2 S donor GYY4137 [12] ( Fig. 1d and Supplementary Fig. S1b ). Moreover, overexpressing CBS in SH-SY5Y cells increases parkin sulfhydration more than eightfold ( Fig. 1e and Supplementary Fig. S1c ). There appears to be negligible basal nitrosylation of parkin present in brain tissue or cell lines, which is unchanged by treatment with H 2 S donors or generating enzymes ( Supplementary Fig. S1d-g ). H 2 S enhances parkin E3 ligase activity via sulfhydration Nitrosylation of parkin decreases its ubiquitination activity both exerted upon itself and on other substrates [3] , [4] . By contrast, in HEK293 cells the H 2 S donor GYY4137 markedly augments parkin autoubiquitination, whereas ‘old’ GYY4137 (GYY4137 exposed to air overnight, to eliminate any H 2 S-donating capacity) fails to influence ubiquitination ( Fig. 2a ). Treatment with GYY4137 results in an increase in parkin E3 ligase activity over time consistent with the activation of parkin via sulfhydration ( Supplementary Fig. S2a ). The stimulation by GYY4137 of parkin’s ubiquitination capacity applies also to proteins that are implicated in the pathogenicity of the disease. AIMP2 expression is elevated in human postmortem brain from both sporadic and familial PD, consistent with the notion that parkin is inactivated in PD and that AIMP2 is neurotoxic [13] , [14] . GYY4137 substantially increases ubiquitination of AIMP2 by parkin ( Fig. 2b ) as well as ubiquitination by parkin of synphilin-1, another parkin substrate implicated in PD ( Fig. 2c ). 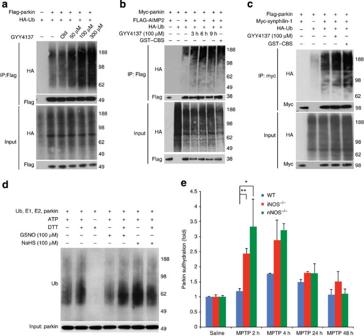Figure 2: Hydrogen sulfide enhances parkin E3 ligase activity via sulfhydration. (a) Parkin E3 ligase activity in HEK293 cells is augmented by GYY4137 in a dose-dependent manner, but not by ‘old’ GYY4137, which was exposed to air overnight in PBS, and is subsequently unable to donate H2S. (b) Parkin activity, measured by target ubiquitination of AIMP2, is stimulated by GYY4137 (100 μM) and by GST–CBS. (c) Ubiquitination by parkin of synphilin-1 is enhanced by treatment with GYY4137 or GST–CBS. (d) Parkin E3 ligase activityin vitrois increased by the addition of 100 μM NaHS and decreased by GSNO. DTT, a reducing agent, returns activity to baseline by reversing sulfhydration or nitrosylation. (e) MPTP influences parkin sulfhydration. Parkin sulfhydration was determined by the maleimide technique in wild-type (WT), nNOS−/−and iNOS−/−mice injected with saline or MPTP, and killed at 2, 4, 24 and 48 h after MPTP injection. Following MPTP treatment, parkin sulfhydration in WT mice increases by almost twofold at 4 h before returning to baseline. Sulfhydration levels are substantially greater at 2–4 h in iNOS and nNOS mice (n=3 mice for each data point). Statistical significance is as noted **P<0.01 and *P<0.05 by the ANOVA analysis, with Tukey HSDpost-hoctest. All data expressed as mean±s.e.m. Figure 2: Hydrogen sulfide enhances parkin E3 ligase activity via sulfhydration. ( a ) Parkin E3 ligase activity in HEK293 cells is augmented by GYY4137 in a dose-dependent manner, but not by ‘old’ GYY4137, which was exposed to air overnight in PBS, and is subsequently unable to donate H 2 S. ( b ) Parkin activity, measured by target ubiquitination of AIMP2, is stimulated by GYY4137 (100 μM) and by GST–CBS. ( c ) Ubiquitination by parkin of synphilin-1 is enhanced by treatment with GYY4137 or GST–CBS. ( d ) Parkin E3 ligase activity in vitro is increased by the addition of 100 μM NaHS and decreased by GSNO. DTT, a reducing agent, returns activity to baseline by reversing sulfhydration or nitrosylation. ( e ) MPTP influences parkin sulfhydration. Parkin sulfhydration was determined by the maleimide technique in wild-type (WT), nNOS −/− and iNOS −/− mice injected with saline or MPTP, and killed at 2, 4, 24 and 48 h after MPTP injection. Following MPTP treatment, parkin sulfhydration in WT mice increases by almost twofold at 4 h before returning to baseline. Sulfhydration levels are substantially greater at 2–4 h in iNOS and nNOS mice ( n =3 mice for each data point). Statistical significance is as noted ** P <0.01 and * P <0.05 by the ANOVA analysis, with Tukey HSD post-hoc test. All data expressed as mean±s.e.m. Full size image To ascertain whether the influence of H 2 S upon ubiquitination is exerted in a direct fashion, we conducted experiments in vitro comparing actions of the NO donor S-nitrosoglutathione (GSNO) and the H 2 S donor NaHS ( Fig. 2d ). As reported previously, GSNO substantially diminishes parkin’s autoubiquitination, [3] whereas such autoubiquitination is markedly augmented by treatment with NaHS. The contrasting actions of H 2 S and NO upon parkin’s ubiquitination activity suggest that the two gasotransmitters may exert reciprocal actions in the pathophysiology of PD. Sulfhydration and nitrosylation typically take place upon the same cysteines in proteins. This suggests that reciprocity between sulfhydration and nitrosylation of parkin impacts pathogenic features of PD. To examine this possibility, we monitored sulfhydration of parkin in brains of mice treated with the neurotoxin MPTP (1-methyl-4-phenyl-1,2,3,6-tetrahydropyridine), which selectively damages dopamine neurons and is often employed as a model for PD ( Fig. 2e and Supplementary Fig. S3a-c ). We noted increased sulfhydration of parkin 2–4 h following MPTP treatment. In brains of mice with targeted deletion of inducible NO synthase (iNOS) or neuronal synthase (nNOS), in which parkin nitrosylation is lost, [3] its sulfhydration is increased by 2.5- to 3-fold. This implies that sulfhydration and nitrosylation of parkin occur reciprocally, presumably on the same cysteines. Parkin sulfhydration enhances its protective functions To ascertain the pathophysiological relevance of reciprocal nitrosylation/sulfhydration of parkin, we sought to identify the sites of sulfhydration. High-resolution electrospray ionization mass spectrometry (MS) technique was implemented, which can differentiate sulfhydration from sulfinic acid oxidation of the cysteine residues. Mass spectrometric analysis revealed five sites of parkin sulfhydration at cysteines 59, 95, 182, 212 and 377 ( Fig. 3a and Supplementary Fig. S4 ). At least one of these sites, cysteine 95, has been identified as being nitrosylated (Harry Ischiropoulos, personal communication). To determine the relative importance of these sites in mediating regulation of parkin ubiquitination activity by H 2 S, we performed systematic mutations of the various cysteines and assessed their activities ( Fig. 3b ). Parkin with C212S or C377S mutations fails to express or is unstable, and could not be evaluated. Enhanced ubiquitination activity of parkin in response to GYY4137 is abolished with C95S mutations, whereas substantial diminution of the enhancement of ubiquitination is evident with C59S and C182S mutations. 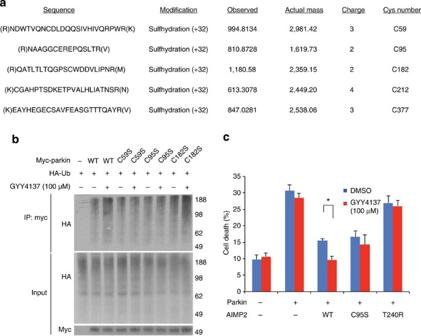Figure 3: Parkin sulfhydration at specific cysteine residues enhances its protective functions. (a) Mass spectrometry detects parkin cysteines sulfhydrated by H2S donor NaHS. (b) C59S, C95S and C182S mutations all substantially reduce parkin activity stimulation by H2S in HEK293 cells. (c) Cell death as monitored by trypan blue exclusion assay in tet-repressible AIMP2-expressing PC12 cells is prevented by parkin overexpression and by GYY4137, whose protective effect is not evident in the absence of parkin, with parkin–C95S or with the T240R catalytically inactive parkin mutant.n=3–6 with *P<0.01 by one-way analysis of variance. All data expressed as mean±s.e.m. Figure 3: Parkin sulfhydration at specific cysteine residues enhances its protective functions. ( a ) Mass spectrometry detects parkin cysteines sulfhydrated by H 2 S donor NaHS. ( b ) C59S, C95S and C182S mutations all substantially reduce parkin activity stimulation by H 2 S in HEK293 cells. ( c ) Cell death as monitored by trypan blue exclusion assay in tet-repressible AIMP2-expressing PC12 cells is prevented by parkin overexpression and by GYY4137, whose protective effect is not evident in the absence of parkin, with parkin–C95S or with the T240R catalytically inactive parkin mutant. n =3–6 with * P <0.01 by one-way analysis of variance. All data expressed as mean±s.e.m. Full size image To determine whether sulfhydration of parkin regulates pathogenic events associated with PD, we monitored cell death using trypan blue exclusion as well as MTT (3-(4,5-dimethylthiazol-2-yl)-2,5-diphenyltetrazolium bromide) assays in PC12 cells overexpressing AIMP2, whose ubiquitination and destruction are elicited by parkin in cellular models of PD [15] ( Fig. 3c and Supplementary Fig. S5a ). Overexpression of AIMP2 triples cell death, whereas parkin overexpression reverses this cytotoxicity. GYY4137 markedly reduces cell death in the parkin-treated cells but not in those overexpressing AIMP2 in the absence of parkin. The selective action of GYY4137 indicates that its cytoprotective effects reflect modifications of parkin rather than some generalized antioxidant influence. This conclusion is supported by GYY4137’s lack of cytoprotective influence in cells overexpressing AIMP2 along with catalytically inactive parkin-T240R. Further evidence that GYY4137 protects by enhancing parkin sulfhydration comes from experiments in which the cytoprotective action of GYY4137 is lost in cells overexpressing parkin–C95S, which is not activated by sulfhydration. Furthermore, we utilized the MPP+ model of PD in PC12 and SH-SY5Y cells in which H 2 S donors provide significant protection against MPP+ toxicity, and inhibition of the H 2 S-producing enzymes results in enhanced toxicity of MPP+, which is relieved by administration of H 2 S donors ( Supplementary Fig. S5b,c ). To resolve whether the antioxidant properties of H 2 S-releasing agents were partially responsible for the neuroprotective effects seen in the AIMP2-overexpressing cells, we determined reactive oxygen species levels in these cells overexpressing vector or various parkin mutants ( Supplementary Fig. 6 ). The various parkin cysteine–serine mutants exhibited increased reactive oxygen species levels as described previously [16] . However, there was not a significant difference in the GYY4137-treated samples at the concentrations that were employed, suggesting that this is not the primary mechanism of protection seen in the experiments described in Fig. 3c . Decreased sulfhydration and increased nitrosylation in PD The pronounced cytoprotective action of parkin sulfhydration as well as the reciprocal relationship of parkin’s nitrosylation and sulfhydration suggest that alterations of sulfhydration participate in the pathophysiology of PD. In accordance, we monitored sulfhydration and nitrosylation in the striatum of PD patients ( Fig. 4 and Supplementary Fig. 7 ). We confirm the increase of parkin nitrosylation in PD brain, [3] and also observe a 60% decrease in parkin sulfhydration in patient brain. 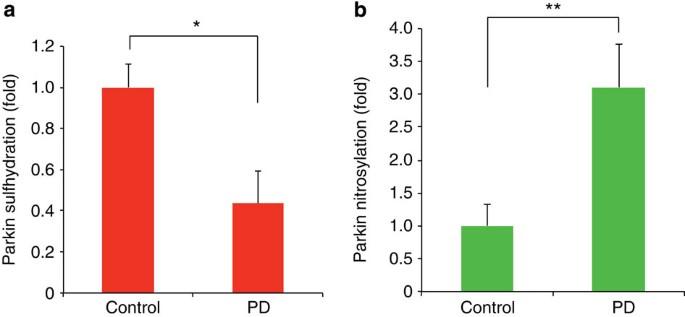Figure 4: Parkin sulfhydration is decreased in PD brain, whereas nitrosylation is increased in PD. (a) The maleimide technique demonstrates that parkin sulfhydration is depleted in the striatum of PD patients. (b) Nitrosylation of parkin is increased in PD patient brain. *P<0.02 by one-way analysis of variance (ANOVA;n=7 control andn=6 PD samples for (a)); **P<0.01 by one-way ANOVA (n=5 each control and PD for (b)). All data are expressed as mean±s.e.m. Figure 4: Parkin sulfhydration is decreased in PD brain, whereas nitrosylation is increased in PD. ( a ) The maleimide technique demonstrates that parkin sulfhydration is depleted in the striatum of PD patients. ( b ) Nitrosylation of parkin is increased in PD patient brain. * P <0.02 by one-way analysis of variance (ANOVA; n =7 control and n =6 PD samples for ( a )); ** P <0.01 by one-way ANOVA ( n =5 each control and PD for ( b )). All data are expressed as mean±s.e.m. Full size image In the present study, we have demonstrated that parkin is physiologically sulfhydrated, a process that enhances its ubiquitination activity. This contrasts markedly with nitrosylation, which decreases such activity. Sulfhydration and nitrosylation of parkin appear to be reciprocal events. This may be related to the difference in chemical reactivity between the two modifications. Nitrosylated cysteines will present a distinctly different chemical group to the local environment than will sulfhydration. In patient striatum, we demonstrate major decreases in parkin sulfhydration, which are reciprocal to the increases in nitrosylation. What might be the comparative roles of parkin nitrosylation and sulfhydration in the pathophysiology of PD? One possibility is that the cell stress of PD leads to increased generation of NO, which accounts for the augmented nitrosylation of parkin in patient brain. Cell stressors do lead to activation of both iNOS and nNOS, and increased S-nitrosylation of several proteins, such as parkin, protein-disulfide isomerase and XIAP, has been speculated to impact PD [17] , [18] , [19] . However, increased NO formation in PD has not been directly demonstrated, and measurements of H 2 S generation in PD are lacking. Nitrosylation and sulfhydration are sensitive and specific reflections of the presence of ambient NO and H 2 S, respectively, implying that altered nitrosylation/sulfhydration in PD brain reflects changes in levels of the two gasotransmitters. Our experiments also establish cytoprotective actions of H 2 S donors, which appear to reflect sulfhydration of parkin. Mutation of C95, a principal site of parkin sulfhydration, largely prevents the protective influences of H 2 S donors, indicating that the donors act via parkin sulfhydration to enhance its ubiquitination activity. C182 and C59 also appear to contribute to influences of H 2 S donors upon parkin. We could not evaluate effects of H 2 S on C212 and C377, as they did not express or were unstable in our cell lines. Interestingly, C95 occurs in human but not rodent parkin, whereas the other sulfhydrated cysteines are conserved in rodent and human species. The beneficial effects of H 2 S donors in PD models may have therapeutic implications. H 2 S donors have already been noted to be beneficial in rodent models of PD [20] , [21] , [22] , and an H 2 S-donating variant of L -3,4-dihydroxyphenylalanine has shown promising effects in cellular models of PD [23] . These influences had been speculated to reflect general antioxidant and anti-inflammatory actions of H 2 S. However, numerous studies have failed to reveal a beneficial effect of antioxidants in PD [24] , [25] . Our findings provide a specific molecular mechanism whereby H 2 S therapy may benefit PD and can explain the ineffectiveness of generalized antioxidant treatment. Modifications of parkin and other interactors of parkin may offer promise in the therapy of PD [15] , [26] , [27] so that H 2 S donors selectively targeted to parkin may provide notable benefit. Generation of plasmids The full-length parkin complementary DNA was cloned into pRK5-myc and pCMV-FLAG (Stratagene) vectors between the Sal I and Not I sites. Full-length cDNAs of synphilin-1 and AIMP2 were cloned into pRK5-myc vector and pCMV-FLAG, respectively, between the Sal I and Not I sites. The cDNA of ubiquitin was cloned into pRK5-HA vector between the Sal I and Not I sites. The generation of C–S mutants was done using the pRK5-myc-parkin construct and site-directed mutagenesis. The integrity of the constructs was confirmed by sequencing. Modified biotin switch assay A modified version of the modified biotin switch assay as described in ref. 9 was used. In brief, overexpressed myc-parkin was transfected into HEK293 cells with polyfect (Qiagen) for 24 h. Cells were treated with 100 μM NaHS (Sigma) as indicated, and were collected in HEN buffer with 1% triton and spun down at 14,000 g for 15 min. The supernatant is then added to lysis buffer plus 2% SDS and 10 mM NEM (N-Ethyl Maleimide) for 1 h at 37 °C while shaking. Blocked proteins are acetone-precipitated with acetone (−20 °C) to remove free NEM, followed by 1 mM dithiothreitol (DTT) treatment for 1 h at 25 °C while shaking. Another round of acetone precipitation was performed to remove the DTT and reduced S-NEM from sulfhydrated residues followed by treatment with 200 μM biotin–NEM for 1 h at 25 °C, which was further followed by precipitation with neutravidin (Thermo Scientific) beads and subsequent analysis via western blot with anti-myc antibody. Maleimide assay Maleimide assay was performed as described in ref. 11 . In brief, cells or tissue were lysed in 20 mM Tris-HCl pH 7.5, 0.1% triton and 100 mM NaCl, and were immunoprecipitated with parkin antibody (Cell Signaling) or other appropriate antibody for 16 h at 4 °C, followed by washing 5 × with lysis buffer plus 300 mM NaCl (wash buffer). Beads were then incubated with 5 μM Red-Maleimide for 2 h at 4 °C while rotating, followed by washing 3 × with wash buffer. Beads were then divided equally between two tubes, with one tube receiving 1 mM DTT and the other tube receiving buffer, and both were rotated for 2 h at 4 °C, followed by washing 3 × with wash buffer. Fifty microlitre of 2 × LDS (Invitrogen) was then added, the beads were boiled for 2 min and proteins were separated on SDS–PAGE and visualized on the LiCor fluorescent scanner. If the two-colour maleimide assay was used, an additional labelling step was included; after incubation with Red-Maleimide and subsequent wash, 1 mM ascorbate was added for 2 h followed by treatment with Green-Maleimide for 2 h and subsequent wash. Beads were then split equally again and treated with DTT as described above. Western blot analysis with the appropriate antibody was performed to ensure that any differences between bead allocations between tubes were taken into account for the experiment. In vitro ubiquitination assay Reactions were performed in a 20-μl mixture containing 50 mM HEPES, pH 7.5, 1 mM MgCl 2 , 1 mM ATP, 1 mM biotin–ubiquitin (BostonBiochem), 110 ng of E1 (BostonBiochem), 900 ng of UbcH7 (BostonBiochem) and His6-Parkin (1.5 μg) that had been treated with either 100 μM of GSNO or NaHS (as indicated) for 20 min before the addition of buffer or 1 mM DTT (as indicated). After 30 min, this was added to the main reaction, which was carried out in darkness and devoid of any reducing agents, such as DTT, at 37 °C (except where specified). After 1 h, the reactions were terminated with an equal volume of 2 × SDS sample buffer, and the products were subjected to western blot analysis with anti-ubiquitin antibody (Cell Signaling). Ubiquitination assay HEK293 cells were transfected with 4 μg of plasmids. After 24 h, the cells were treated with the MG132 (Sigma) followed by the selected drugs (as indicated) for the specified time course (3–9 h). If cells were transfected with CBS, 500 μM of L -cysteine was added to the media as a supplement for H 2 S generation. After 2–9 h, all samples were collected together to ensure that all samples were treated with MG132 for equal time and only the time treated with H 2 S varied. The cells were collected by washing with cold PBS and then lysed with immunoprecipitation buffer (25 mM HEPES, pH 7.5, 100 mM NaCl, 0.5% triton X-1000, 1 mM EDTA, Roche Complete Protease Inhibitor Tablet). The lysates were then sonicated at 4 °C for 10 s and rotated for 15 min at 4 °C, followed by centrifugation at 14,000 g for 15 min. The supernatants were combined with 30 μl EZ-View anti-myc or anti-FLAG (Sigma) beads overnight at 4 °C. The beads were pelleted and washed five times using immunoprecipitation buffer with 500 mM NaCl. The precipitates were resolved on SDS–PAGE gel and subjected to western blot analysis with antibodies against myc or HA (Roche). Bands were visualized with chemiluminescence (Pierce). Animals and treatment All experiments were approved and conformed to the guidelines set by the Institutional Animal Care Committee. Ten-week-old iNOS-deficient mice and nNOS-deficient mice (Jackson Laboratories) and their wild-type counterparts were used. Mice received four intraperitoneal injections of MPTP–HCl (20 mg kg −1 of free base; Sigma) in saline at 2 h intervals in 1 day, and were killed at selected time points as indicated after the last injection. Control mice received saline only. The mouse brains were collected and S-sulfhydration of parkin in the whole brain was determined by maleimide assay. Human tissue Human brain tissue was obtained through the brain donation programme of the Morris K. Udall Parkinson’s Disease Research Center at the Johns Hopkins Medical Institutions according to Health Insurance Portability and Accountability regulations. This research proposal involves anonymous autopsy material that lacks identifiers of gender, race or ethnicity. The Johns Hopkins Medical Institutions joint committee on clinical investigations decided that the studies in this proposal are exempt from human subjects approval because of federal register 46.101 exemption number 4. Seven age-matched control brains, and six PD and/or DLBD brains were utilized for the detection of S-sulfhydration and S-nitrosylation of parkin by the maleimide assay. AIMP2-inducible cell lines As described previously, PC12 cells were grown in DMEM containing 10% horse serum, 5% No-Tet fetal bovine serum in a 5% CO 2 atmosphere [15] . Tet-off cells (Clontech) were used to create PC12 cell lines expressing inducible AIMP2 as described previously. Differentiation was initiated by the addition of 100 ng ml −1 NGF to the culture medium. NGF was replenished daily for differentiation. Cell-viability analysis AIMP2-inducible PC12 cells were plated in a six-well plate for viability. Cells were transfected with indicated plasmids using Lipofectamine 2000 (Invitrogen) according to the manufacturer’s instructions. Cells were incubated with 100 μM GYY4137 or vehicle after 2 days of induction and differentiation with NGF. To assess cell viability in the PC12 cell experiments, we used the trypan blue exclusion assay. Cells were resuspended in plating medium with trypan blue stain for 5 min. We counted the percentage of blue-stained cells among total cells using the Cell Countess cell counter to determine a percentage of cell death in the trypan blue exclusion assay described previously [10] . The MTT assay was also used to determine cell viability. Briefly, cells were incubated with MTT for 2 h, after which the supernatant was removed and centrifuged to collect any floating cells. One millilitre of dimethylsulfoxide was used to lyse the remaining cells, after which any pelleted cells were lysed with 1 ml of dimethylsulfoxide and added to the original well from which it was taken. This was incubated at room temperature for 20 min while shaking. Absorbance measurements were then taken at 570 and 630 nm to determine cell viability. Statistical analysis All data are expressed as mean±s.e.m. Statistical significance between sample sets was analysed by analysis of variance with post-hoc test where appropriate. Mass spectral analysis Purified His6-Parkin (BostonBiochem) was again purified with spin column to remove any trace DTT, followed by incubation in 50 mM HEPES and 100 mM NaCl buffer with 100 μM NaHS for 1 h. These samples were then digested with trypsin and run on high-resolution tandem mass spectrometry array for analysis. Database searching for tandem mass spectra were extracted, charge state deconvoluted and deisotoped by 1 version 3. All MS/MS samples were analysed using Mascot (Matrix Science, London, UK; version Mascot) and Sequest. Mascot was set up to search the NCBInr_20080819 database (selected for Homo sapiens , 2, 133,769 entries) assuming the digestion enzyme trypsin. Mascot was searched with a fragment ion mass tolerance of 0.050 Da and a parent ion tolerance of 15 p.p.m. Oxidation of methionine, persulfide of cysteine, sulfur dioxide of cysteine (sulfination), sulfitolysis of cysteine, N-ethylmaleimide on cysteines of cysteine, N-ethylmaleimide hydrolysis of cysteine, NEM+S (NEM-modified sulfhydration) of cysteine and NEM+S+H 2 O of cysteine were specified in Mascot as variable modifications. Criteria for protein identification, Scaffold (version Scaffold_3.4.3, ProteomeSoftware Inc., Portland, OR), was used to validate MS/MS-based peptide and protein identifications. Peptide identifications were accepted if they could be established at greater than 95% probability as specified by the Peptide Prophet algorithm [28] . Protein identifications were accepted if they could be established at greater than 95% probability and contained at least two identified peptides. Protein probabilities were assigned by the Protein Prophet algorithm. [29] Proteins that contained similar peptides and could not be differentiated based on MS/MS analysis alone were grouped to satisfy the principles of parsimony. How to cite this article: Vandiver, M.S. et al . Sulfhydration mediates neuroprotective actions of parkin. Nat. Commun. 4:1626 doi: 10.1038/ncomms2623 (2013).